Increased sensitivity to climate change in disturbed ecosystems Human domination of the biosphere includes changes to disturbance regimes, which push many ecosystems towards early-successional states. Ecological theory predicts that early-successional ecosystems are more sensitive to perturbations than mature systems, but little evidence supports this relationship for the perturbation of climate change. Here we show that vegetation (abundance, species richness and species composition) across seven European shrublands is quite resistant to moderate experimental warming and drought, and responsiveness is associated with the dynamic state of the ecosystem, with recently disturbed sites responding to treatments. Furthermore, most of these responses are not rapid (2–5 years) but emerge over a longer term (7–14 years). These results suggest that successional state influences the sensitivity of ecosystems to climate change, and that ecosystems recovering from disturbances may be sensitive to even modest climatic changes. A research bias towards undisturbed ecosystems might thus lead to an underestimation of the impacts of climate change. In climate change experiments, the vegetation at a study site is typically viewed as a system that is stable or close to equilibrium. A common objective is to assess whether a climatic treatment can push the system away from this hypothesized stable state. Most ecosystems, however, are not in equilibrium. Rather, they change over time and are often recovering from past disturbances [1] . This is particularly true today, as increasing human domination of the biosphere [2] pushes many ecosystems towards a more dynamic, early-successional state. Although Odum [3] suggested in 1969 that early-successional ecosystems are more sensitive to perturbation than late-successional ones, this feature of ecosystems is rarely taken into account in climate change research. Single-site climate change experiments have reported that disturbed or recovering systems were sensitive to climate manipulations [4] , [5] , but it remains unclear whether an ecosystem’s dynamic state determines its sensitivity to climatic changes. Grime et al . [4] found that a stable, late-successional grassland was more resistant to the same climatic manipulations than a dynamic, early-successional grassland. Several authors have suggested that successional state and disturbance history could modulate responses to climatic change [6] , [7] , but a lack of data has prevented direct investigations of these relationships. In addition to the experimental field manipulation of climatic conditions, two other major field-based approaches can assess the effects of climate change on ecosystems: long-term observations [8] , [9] and multi-site and gradient studies across climatically different regions [10] , [11] . Each approach has its own merits and limitations [7] , [12] , but the combination of these approaches can be particularly valuable. For example, contrasting results from experiments conducted in different climatic regions may highlight shifting sensitivities, such as a positive warming effect on aboveground biomass in cold regions and negative effects in water-limited regions [13] , [14] , [15] . Also, long-term experiments have often detected an altered pattern of response over time, including linear increases [16] , dampening [17] , [18] and reversals [19] , [20] . Despite the added value of combined approaches, long-term multi-site experiments are rare. Shrublands constitute an important component of global and European terrestrial vegetation [21] , [22] , provide multiple ecosystem services [23] and are strongly affected by ongoing environmental changes. The encroachment of shrubs has been observed in many arid and semiarid regions of the world, mostly attributed to changes in land use [24] . Expanding shrublands and other types of woody vegetation have been estimated to be among the largest carbon sinks in the United States [25] . As long-lived woody plants, shrubs differ from herbaceous plants in their life history, ecophysiology, biomass allocation and sensitivity to disturbance, suggesting a potentially different sensitivity to changing climate. A global meta-analysis found that shrubs respond to warming more strongly than other woody and herbaceous plants [13] . All these considerations suggest that shrubs and shrublands deserve special attention in climate change impact research. Here we investigated the responses of vegetation (abundance, species richness and species composition) to experimental warming and drought in a standardized field experiment across seven shrubland sites in Europe over 7–14 years ( Fig. 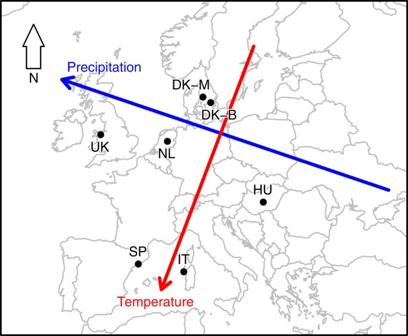Figure 1: Location of the climatic manipulation experiments in Europe. Arrows depict the broad-scale gradients in precipitation and temperature. DK-B, Denmark at Brandbjerg; DK-M, Denmark at Mols; HU, Hungary; IT, Italy; NL, Netherlands; SP, Spain; UK, United Kingdom. 1 ; Table 1 ; www.increase.ku.dk ; UK: United Kingdom, NL: The Netherlands, DK-M and DK-B: Denmark, HU: Hungary, SP: Spain, IT: Italy ). Our results show that the studied shrublands are generally quite resistant to long-term experimental warming and drought, with no across-site responses and few responses within individual sites. However, sites that respond to treatments are all recovering from disturbance; vegetation does not respond to treatments in sites that are in a steady state (as assessed by long-term trend in vegetation abundance in the control plots at each site). This suggests that sensitivity to climate change may be related to the successional state of ecosystems, and that ecosystems recovering from disturbances may be sensitive to even modest climatic changes. Figure 1: Location of the climatic manipulation experiments in Europe. Arrows depict the broad-scale gradients in precipitation and temperature. DK-B, Denmark at Brandbjerg; DK-M, Denmark at Mols; HU, Hungary; IT, Italy; NL, Netherlands; SP, Spain; UK, United Kingdom. Full size image Table 1 Characteristics of the study sites. Full size table Responses to warming and drought treatments Neither warming nor drought affected total vegetation abundance or species richness across all sites averaged after 7–14 years of experimental manipulation (long-term responses) ( Figs 2 and 3 ). We found that, across sites, the change in vegetation composition was marginally affected by both warming ( P =0.061; Fig. 4a ) and drought ( P =0.072; Fig. 4b ). Within the individual sites, warming decreased species richness at SP but had no significant effect on the other vegetation parameters at any of the sites ( Figs 2a , 3a and 4a ). Drought decreased total cover at NL ( P =0.02; Fig. 2b ) and species richness at SP ( P =0.001; Fig. 3b ). Drought also induced a greater vegetation change at DK-M ( P =0.011) and SP ( P =0.044) than in the respective control plots ( Fig. 4b ). 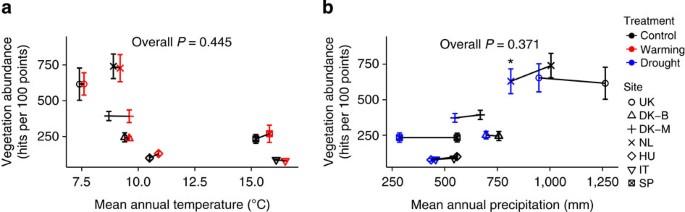Figure 2: Change in vegetation abundance in response to treatments. Total vegetation abundance at the seven sites 7–14 years after the start of the experiments in the warming (a) and drought (b) treatments. * indicates a significant difference (P<0.05) between treated and control plots; linear mixed model (mean±s.e.,n=3). DK-B, Denmark at Brandbjerg; DK-M, Denmark at Mols; HU, Hungary; IT, Italy; NL, Netherlands; SP, Spain; UK, United Kingdom. Figure 2: Change in vegetation abundance in response to treatments. Total vegetation abundance at the seven sites 7–14 years after the start of the experiments in the warming ( a ) and drought ( b ) treatments. * indicates a significant difference ( P <0.05) between treated and control plots; linear mixed model (mean±s.e., n =3). DK-B, Denmark at Brandbjerg; DK-M, Denmark at Mols; HU, Hungary; IT, Italy; NL, Netherlands; SP, Spain; UK, United Kingdom. 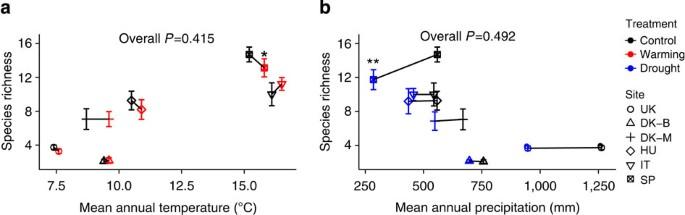Figure 3: Change in species richness in response to treatments. Species richness at six sites 7–14 years after the start of the experiments in the warming (a) and drought (b) treatments. * (P<0.05) and ** (P<0.01) indicate significant differences between treated and control plots; linear mixed model (mean±s.e.,n=3). NL was omitted from this analysis due to its single-species vegetation. DK-B, Denmark at Brandbjerg; DK-M, Denmark at Mols; HU, Hungary; IT, Italy; SP, Spain; UK, United Kingdom. Full size image Figure 3: Change in species richness in response to treatments. Species richness at six sites 7–14 years after the start of the experiments in the warming ( a ) and drought ( b ) treatments. * ( P <0.05) and ** ( P <0.01) indicate significant differences between treated and control plots; linear mixed model (mean±s.e., n =3). NL was omitted from this analysis due to its single-species vegetation. DK-B, Denmark at Brandbjerg; DK-M, Denmark at Mols; HU, Hungary; IT, Italy; SP, Spain; UK, United Kingdom. 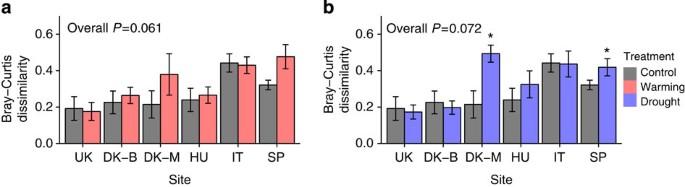Figure 4: Change in vegetation composition in control and treated plots. Bray–Curtis dissimilarity between pretreatment year and 7–14 years after the start of the experiments in the warming (a) and drought (b) treatments. * indicates a significant difference (P<0.05) between treated and control plots; linear mixed model. NL was omitted from this analysis due to its single-species vegetation (mean±s.e.,n=3). DK-B, Denmark at Brandbjerg; DK-M, Denmark at Mols; HU, Hungary; IT, Italy; SP, Spain; UK, United Kingdom. Full size image Figure 4: Change in vegetation composition in control and treated plots. Bray–Curtis dissimilarity between pretreatment year and 7–14 years after the start of the experiments in the warming ( a ) and drought ( b ) treatments. * indicates a significant difference ( P <0.05) between treated and control plots; linear mixed model. NL was omitted from this analysis due to its single-species vegetation (mean±s.e., n =3). DK-B, Denmark at Brandbjerg; DK-M, Denmark at Mols; HU, Hungary; IT, Italy; SP, Spain; UK, United Kingdom. Full size image We found even fewer responses when we performed the same set of analyses for years 2–5 after onset of the experimental manipulation (short-term responses; Supplementary Figs 1–3 ). Warming increased total vegetation abundance at the cross-site level ( P =0.035; Supplementary Fig. 1 ), but this effect disappeared in the long term ( Supplementary Fig. 4a ). The only individual-site level response to appear over the short term occurred at SP, where drought reduced species richness ( P =0.011). In the four additional site-level variables that displayed long-term (but not short-term) responses, effect sizes increased over time ( Supplementary Fig. 4 ). The effect of the dynamic state on vegetation sensitivity To quantify the dynamic state of the sites, we investigated the change in vegetation abundance in the control plots during the study period. Total vegetation abundance significantly increased over time in the control plots at NL (6.3% per year; P <0.01), SP (3.8% per year; P <0.01) and DK-M (2.7% per year; P <0.01), but did not change significantly at the other four sites ( Fig. 5 ). The climatic manipulations thus led to significant responses only at sites (NL, SP and DK-M) that showed significant successional changes in the control plots. In addition, the dynamic state of the sites (as assessed by the trend in vegetation abundance in the control plots) was related to treatment responses of the vegetation (effect sizes of the treatment effects on Bray–Curtis dissimilarity) for both warming ( P =0.04) and, marginally, drought ( P =0.07; Fig. 6 ). In contrast, these effect sizes of the warming and drought treatments were not related to mean annual temperature (MAT; P =0.57 and 0.97, respectively) or mean annual precipitation (MAP; P =0.36 and 0.43, respectively) at the sites. 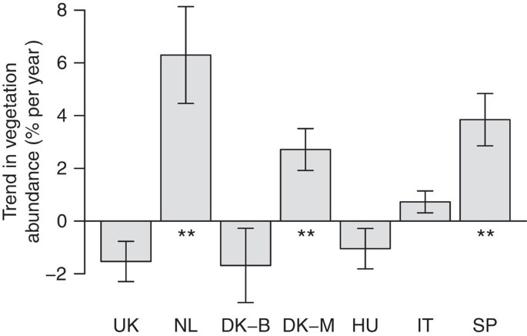Figure 5: Change in total cover in the control plots over the experimental period. Average annual change in total cover (TC) in the control plots during the study period, estimated by linear regression of TC over time (**P<0.01). Yearly cover change is expressed relative to the cover of the pretreatment year (% of pretreatment year cover). Error bars are the s.e. of the estimated trends (ndiffers per country and ranges from three replicates times seven years (21 data points) to three replicates times 15 years (45 data points); see the Methods). DK-B, Denmark at Brandbjerg; DK-M, Denmark at Mols; HU, Hungary; IT, Italy; NL, Netherlands; SP, Spain; UK, United Kingdom. Figure 5: Change in total cover in the control plots over the experimental period. Average annual change in total cover (TC) in the control plots during the study period, estimated by linear regression of TC over time (** P <0.01). Yearly cover change is expressed relative to the cover of the pretreatment year (% of pretreatment year cover). Error bars are the s.e. of the estimated trends ( n differs per country and ranges from three replicates times seven years (21 data points) to three replicates times 15 years (45 data points); see the Methods). DK-B, Denmark at Brandbjerg; DK-M, Denmark at Mols; HU, Hungary; IT, Italy; NL, Netherlands; SP, Spain; UK, United Kingdom. 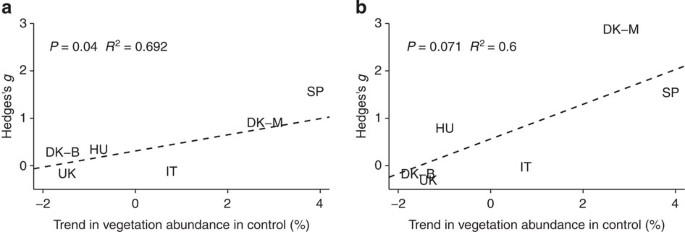Figure 6: Relationships between effect size of vegetation change in response to treatments and successional tendency of the sites. Relationships between the effect size (Hedges’sg) of warming (a) and drought (b) effects on changes in vegetation composition relative to the start of the experiment (assessed by Bray–Curtis dissimilarity) and the successional tendency (calculated as the trend in total cover (relative to pretreatment total cover) in the control plots). ThePvalues represent the significance of the linear regressions. DK-B, Denmark at Brandbjerg; DK-M, Denmark at Mols; HU, Hungary; IT, Italy; SP, Spain; UK, United Kingdom. Full size image Figure 6: Relationships between effect size of vegetation change in response to treatments and successional tendency of the sites. Relationships between the effect size (Hedges’s g ) of warming ( a ) and drought ( b ) effects on changes in vegetation composition relative to the start of the experiment (assessed by Bray–Curtis dissimilarity) and the successional tendency (calculated as the trend in total cover (relative to pretreatment total cover) in the control plots). The P values represent the significance of the linear regressions. DK-B, Denmark at Brandbjerg; DK-M, Denmark at Mols; HU, Hungary; IT, Italy; SP, Spain; UK, United Kingdom. Full size image While the cross-site pattern of responses we found suggested an important and rarely explored relationship between recovery from disturbance and sensitivity to climate, we found that vegetation in most sites was resistant to treatments, and site-specific outcomes were consistent with results from other ecosystems. The negative response of total vegetation abundance to drought at NL is similar to findings in other studies [4] , [26] , including a meta-analysis [10] . Note that vegetation abundance was increasing at this site ( Fig. 5 ); thus, the negative drought effect does not imply a decline but rather a reduced increase. The negative effect of drought on species richness at SP agrees with other studies in semiarid systems [26] , and is most likely related to reduced colonization due to water stress. The fact that compositional change was the parameter with most of the significant responses (two sites) suggests that plant community composition is among the most sensitive ecosystem properties to climatic change, and can respond even when ecosystem characteristics like total vegetation abundance are unaffected [27] . This fits the pattern previously suggested in a hierarchical response framework [28] . Most responses detected in the long term (7–14 years) were not present in the short term (2–5 years), and effect sizes increased over time. Although an increasing effect size over time has been found before [16] , another study [17] lists examples of effects fading within 10 years due to acclimation, species reordering or new limiting factors. It has also been found that short-term changes in community composition can be reversed within a few years due to species interactions [19] , [20] . This volatility highlights the risk in basing conclusions on short-term studies. Although we found a few site-level responses, the overall resistance of the studied shrublands to 7–14 years of experimental warming and drought is noteworthy. Resistance to long-term climatic manipulation has been reported for various ecosystems, such as arctic tundra [29] , tall-grass steppe [30] , calcareous grassland [31] and arid shrubland [32] , indicating a generally widespread ecosystem resistance to climatic change. The lack of responses to experimental climate change observed in our shrubland ecosystems may be related to the relatively moderate treatment regimes applied (an average 0.43 K increase in temperature and 22% reduction in annual precipitation). However, our treatments are in line with recently observed decadal changes (0.13 K warming [33] ) at a multi-decadal (50 years) timescale and are similar to treatments in many other climate change experiments [6] , [13] , [19] . Although the treatments are not that strong, consistent moderate warming and drought for 8–14 years may be an extreme situation, which is supported by the finding that most responses emerged only in the long run. Experiments that impose larger treatment magnitudes have a greater chance to exceed thresholds and thus may provide important insights into ecosystem sensitivity, but are also more likely to have artefacts. For example, both modelling [34] and experimental studies [35] show that an unrealistic abrupt change in CO 2 concentration overestimates ecosystem sensitivity compared with a gradual change to the same level. Mild treatments, on the other hand, may not immediately push the environment beyond observed levels of interannual variation, but may allow the detection of effects that accumulate slowly or result from interacting factors. In our case, the relatively mild treatments allowed us to detect differences in sensitivity that seem to be related to successional states and disturbance events. All sites that responded to the treatments had vegetation that was increasing in abundance following a disturbance. NL was recovering from a previous cutting-management intervention, SP was recovering from a fire before the start of the experiment and DK-M was affected by a severe outbreak of heather beetles (and consequent mowing) during the first study year (1999). The observed treatment effects at these sites suggest an altered recovery in the drought plots compared with the control plots. In contrast, at the four sites that did not respond to treatments, vegetation abundance did not change over time, suggesting that the vegetation was in a relatively steady state. These results indicate that the dynamic state of ecosystems may be an important predictor of sensitivity to climate change. Disturbances are likely to modulate ecosystem responses to climatic change because different life stages of individual plants and successional stages of plant communities differ in their sensitivity to environmental conditions (for example, drought stress). Regeneration of the previously dominant vegetation after a disturbance can be affected by a climatic change that would hardly affect established mature vegetation because early life stages of plants are often more sensitive to environmental changes than mature plants [36] , [37] , [38] . Changing environmental conditions may not directly lead to an ecosystem state shift, but may just reduce the resilience of an ecosystem (ability to recover from a perturbation), thus making it more prone to state shift, but only when disturbed [39] , [40] . This implies that the resistance of some ecosystems to long-term and severe manipulations of climatic factors, such as a 3 K increase in temperature [31] or a 30% decrease/increase in precipitation [32] , does not necessarily hold after the occurrence of a major natural or anthropogenic disturbance. The results of our study hint that climatic change reduces the resilience of the studied shrubland ecosystems, even though the imposed treatments had few effects in the absence of disturbances. The results of this study highlight the potential importance of successional state, which has mostly been overlooked in climate change studies. There are several important implications for the planning and interpretation of climate change impact research. The sensitivity of an ecosystem to climatic change is likely to be critically determined by its ability to recover after a disturbance. This implies that new experiments should account for site history and quantify successional state or should ideally deliberately include disturbances in the experimental set-up. In addition, meta-analyses should include the dynamic state of study systems. Finally, researchers should recognize that many results from climate change experiments to date come from relatively stable near-natural ecosystems [6] , [7] , [13] ; disturbed, early-successional systems are often avoided. This bias towards relatively stable ecosystems, coupled with the short time frame covered by most studies may lead to a broad underestimation of ecosystem sensitivity to climate change. Study sites We studied seven sites ( Fig. 1 ) that spanned different climatic regions within Europe ( Table 1 ). MAT at the sites ranged from 7.4 to 16.1 °C, and MAP ranged from 544 to 1,263 mm ( Table 1 ). The sites contained the major types of shrubland that occur in temperate Europe: Atlantic heathland (UK, United Kingdom; NL, The Netherlands, DK-M and DK-B, Denmark), continental forest steppe (HU, Hungary), and Mediterranean machia/garrigue (SP, Spain and IT, Italy). The sites were established in 1998 (UK, NL, DK-M and SP), 2001 (HU and IT) or 2004 (DK-B). We used climatic data recorded in the control plots of each experimental site to obtain the climate characteristics of each site. The treatment effect at each site was calculated as the average difference in measured temperature, precipitation and soil moisture between control and treatment plots. Experimental manipulations We used the same experimental technology for the three treatments (warming, drought and control) at each study site. The warming plots received passive warming at night; the plots were automatically covered with curtains that reflected outgoing radiation after sunset [41] . The warming curtains were automatically withdrawn during rain events. The night-time warming approach is in accordance with reports that in the ongoing global warming there is a higher rate of warming during the night than during the day [42] . A study comparing different methods concluded that the passive night-time warming approach is one of the most realistic and applicable [43] . Although the warming effect obtained with this technique is greatest during the night, there is also some carry-over effect into the day [44] . The warming treatment was applied year-round and resulted in an average temperature increase of 0.43 K (range: 0.2–0.9 K, Table 2 ). This is relatively modest but is in line with observed past changes [33] at a multi-decadal (50 years) timescale. Table 2 Experimental manipulations at the study sites. Full size table During rain events, transparent waterproof sheets automatically covered the drought plots, excluding the rain. Note that these sheets covered the drought plots only for the duration of the rain events, thus avoiding warming effects [41] . The timing and duration of the experimental drought differed among the sites, dependent on seasonality and regional climatic predictions ( Table 2 ). We excluded an average of 22% of precipitation (range: 8–49%, Table 2 ), and rain exclusion resulted in an average soil moisture decline of 36% (range 23–47%, Table 2 ) by the end of the drought periods. Control plots had the same metallic scaffolding as the treated plots, but without curtains and sheets. Each treatment had three replicate 20 m 2 plots except at DK-B, which had six replicates and a plot size of 9.1 m 2 . Replicate numbers were limited by logistical and financial constraints associated with such complex field experiments. Replicates were grouped in blocks consisting of a control, a warming and a drought plot. There was no blocking of control and warming plots at the NL site. Sampling of vegetation We used the point-intercept method to measure plant cover and composition. At each site, 300 permanent positions were sampled per plot per sampling year, except for DK-M (200 positions) and DK-B (50 positions per plot in six replicate plots). The points were arranged either along lines (HU, SP, IT and NL) or in grids per experimental plot (DK-M, DK-B and UK). Vegetation sampling was conducted at least 50 cm from the plot edge to avoid edge effects. Pin hits for all vascular plant species were recorded. Only the first hit was recorded at IT where the vegetation was open. The vegetation was sampled annually following the start of the experiments, but the sampling years varied subsequently: UK: 1998–2000, 2002–2003 and 2007–2012; NL: 1998–2003, 2005, 2008, 2009 and 2012; DK-M:1998–2001, 2003, 2006,and 2009–2012; DK-B: 2004 and 2006–2012; HU: 2001–2012; SP: 1999–2012; and IT: 2001–2004 and 2010–2012. We used the number of hits per 100 pins as a proxy for plant or vegetation abundance, as typical in multi-year climate change experiments [26] where the experimental plots are too small for the regular harvesting of biomass. Data analysis The cover of vascular plants for years 7–14 was used to assess the mid- to long-term responses of shrubland plant communities to experimental manipulations. We used linear mixed models from the lme4 package [45] in R [46] to identify treatment effects on total cover, species richness and compositional change. Compositional change was assessed with the Bray–Curtis dissimilarity [47] of the plant community in a specific year compared with the plant community at the beginning of the experiment at the same plot (pretreatment year or first year at SP). The Bray–Curtis dissimilarity was calculated for each plot in all sampling years with the vegdist function in the vegan package [48] in R. Values of total cover, species richness and compositional change were averaged across available years (7–14 for long-term responses and 2–5 years for short-term responses) for each plot to avoid temporal pseudoreplication. We calculated P values for fixed-effect parameters with an analysis of variance using the Satterthwaite estimation of the degrees of freedom with the lmerTest package [49] . We applied separate models to analyse the effects of the warming and drought treatments and used site and site:block as random factors for the cross-site tests; block was a random factor in the site-specific analyses (the warming effect in NL was analysed with a linear model, since warming and control plots were not blocked). Data were log-transformed (ln) to obtain normality and homoscedasticity in the cross-site analyses. NL was excluded from all tests related to species richness and the Bray–Curtis dissimilarity because it only had one vascular plant species. We calculated the effect sizes of the treatments as Hedges’s g [50] : Where μ treatment and μ control are the average values in treatment and control plots. s * is the pooled s.d. of both control and treatment plots, calculated as follows: Where n control and n treatment are the number of replicates and σ 2 control and σ 2 treatment are the variances of control and treatment plots. Finally, J is a factor to correct for bias (related to small sample size) in the estimated effect size: For variables with a significant treatment response in either the short or the long term, we calculated the effect size over time. The successional status of the various sites was determined by linear regression of vegetation abundance (relative to the vegetation abundance at the start of the experiment) in the control plots over time. The slope estimates from these linear regressions (average annual change) were used as a measure of the dynamic status or successional trend for each site, with higher values indicating more dynamic vegetation. We investigated whether the effect size of the variable related to plant community composition (Bray–Curtis dissimilarity) was related to MAT or MAP or the dynamic status of the sites with linear regression. All analyses where done in R [46] . How to cite this article : Kröel-Dulay, G. et al . Increased sensitivity to climate change in disturbed ecosystems. Nat. Commun. 6:6682 doi: 10.1038/ncomms7682 (2015).